Aerosol transmission is an important mode of influenza A virus spread Influenza A viruses are believed to spread between humans through contact, large respiratory droplets and small particle droplet nuclei (aerosols), but the relative importance of each of these modes of transmission is unclear. Volunteer studies suggest that infections via aerosol transmission may have a higher risk of febrile illness. Here we apply a mathematical model to data from randomized controlled trials of hand hygiene and surgical face masks in Hong Kong and Bangkok households. In these particular environments, inferences on the relative importance of modes of transmission are facilitated by information on the timing of secondary infections and apparent differences in clinical presentation of secondary infections resulting from aerosol transmission. We find that aerosol transmission accounts for approximately half of all transmission events. This implies that measures to reduce transmission by contact or large droplets may not be sufficient to control influenza A virus transmission in households. Influenza A viruses are believed to spread between humans through exposure to respiratory droplets expelled during coughing or sneezing from infectious individuals. A distinction is typically made between larger droplets that are believed to settle to ground within 1–2 m, versus smaller droplet nuclei particles with aerodynamic diameter below 5 μm [1] , [2] , [3] , [4] that can remain airborne for longer periods but may desiccate quickly, depending on environmental conditions. These latter particles are also referred to as aerosols and retain infectivity [4] . The relative importance of contact, droplet and aerosol transmission of influenza viruses in humans has not been established, making it difficult to develop evidence-based infection control policies in various settings [5] . Influenza viruses can survive for hours on non-porous surfaces, but are not thought to survive long on hands [6] , [7] . Influenza viral RNA can be detected in the household environment of infected individuals, and hand hygiene can reduce environmental contamination [8] . Hand hygiene has appeared to reduce but not eliminate transmission in some studies but not others [9] , [10] , [11] , [12] , suggesting that contact spread has a partial role in influenza virus transmission. In studies of exhaled breath particles from healthy subjects during tidal breathing, concentrations of particles vary from 1 to >10,000 particles per liter, with the majority <0.3 μm in diameter [13] . Infectious virus and viral RNA can be detected in both larger particles >5 μm and smaller particles <5 μm [14] , [15] , [16] . Experimental studies have demonstrated that influenza virus can remain infectious in small particle aerosols, and can transit across rooms [17] . Influenza viral RNA has been detected in a hospital emergency department [18] and aerosol transmission was implicated in a hospital outbreak of seasonal influenza [19] . These data demonstrate the potential contribution of aerosols to influenza transmission. However, there is limited empirical evidence of aerosol transmission in the literature to date [4] . Ferret studies have provided evidence supporting the various modes of influenza virus transmission [4] , and notably in the 1940, s, one study provided evidence supporting aerosol transmission [20] . Influenza virus infection is associated with a varying spectrum of disease that typically ranges from subclinical or asymptomatic to acute febrile acute respiratory illness [21] , [22] . An important observation from human challenge studies is that aerosolized influenza A viruses are infectious at low doses, and tend to cause more ‘typical influenza-like disease’ (that is, fever plus cough) than intranasal inoculation, which mimics contact and droplet transmission [22] , [23] . Similar observations have also been reported in the ferret model [24] . This could be explained by infection with small particles in the conducting airways or lower respiratory tract, eliciting a more vigorous host response characterized by fever and coughing. This leads to the hypothesis that influenza A virus infections initiated by aerosol transmission could have a different clinical presentation on average than infections by the contact or droplet route, and that aerosol spread would be more likely to manifest in fever plus cough. Differing clinical presentation depending on the primary site of infection is thought to occur for other infectious diseases, for example, smallpox, and Milton suggested the term ‘anisotropic’ for infections with this property [25] . Based on the hypothesis that average clinical presentation differed depending on the mode of transmission, we developed a mathematical model to permit inference on the contribution of each mode to transmission of influenza A virus in households from data from two randomized controlled trials of surgical masks and hand hygiene, in Hong Kong and Bangkok. We found that aerosol transmission accounted for approximately half of all transmission events. This implies that measures to reduce transmission by contact or large droplets may not be sufficient to control influenza A virus transmission in households. Descriptive analysis In total, the studies in Hong Kong and Bangkok included successful follow-up of 275 and 507 index cases with confirmed influenza A, respectively, ( Supplementary Tables S1–S2 ). There was no statistically significant difference between study arms in the risk of confirmed influenza A virus infections in household contacts and initial reports of those studies concluded that these interventions could have had at most a small effect on overall transmission [11] , [12] . In both studies, household contacts with confirmed influenza A virus infection had slightly higher but non-significant risks of fever plus cough in the intervention arms compared with the control arm ( Supplementary Table S3 ). However, when the cumulative incidence of confirmed influenza infections were plotted for household contacts, we identified a change in the risk of fever plus cough that was particularly apparent in the households in Bangkok ( Fig. 1 , Supplementary Fig. S1 ). These changes are consistent with our hypothesis that hand hygiene and face mask interventions would reduce contact and large droplet transmission, increasing the contribution of aerosol transmission in the intervention arms which consequently led to an increased risk of fever plus cough among the confirmed infections in household contacts in the intervention arms. 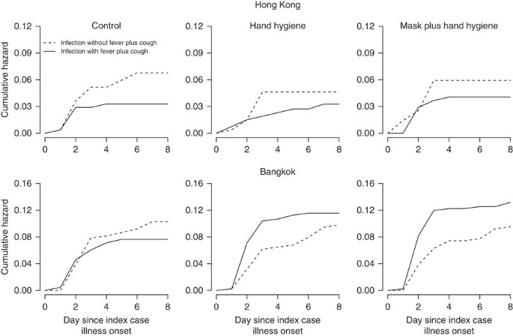Figure 1: Risk of infection and illness in household contacts. Cumulative hazards of confirmed influenza A virus infections presenting with fever plus cough or not presenting with fever plus cough, in household contacts in 275 and 507 households in Hong Kong and Bangkok, respectively. Increases in the risk of confirmed infection with fever plus cough, and decreases in the risk of confirmed infection without fever plus cough, are particularly apparent in the intervention arms compared with the control arm in Bangkok. Figure 1: Risk of infection and illness in household contacts. Cumulative hazards of confirmed influenza A virus infections presenting with fever plus cough or not presenting with fever plus cough, in household contacts in 275 and 507 households in Hong Kong and Bangkok, respectively. Increases in the risk of confirmed infection with fever plus cough, and decreases in the risk of confirmed infection without fever plus cough, are particularly apparent in the intervention arms compared with the control arm in Bangkok. Full size image Modes of transmission Fitting the transmission model to the data from each study, we found that under a wide range of assumed efficacies of hand hygiene and face masks, aerosol spread remained the dominant mode of influenza A virus transmission, with consistency in the estimated contribution to overall transmission between the two settings ( Fig. 2 ). Under a plausible exemplar scenario where randomization to the hand hygiene intervention reduced contact transmission by 50%, although randomization to face masks plus hand hygiene reduced both contact and droplet transmission by 50%, we estimated that in the control arm aerosol transmission contributed to 51% of secondary infections in Hong Kong and 42% of secondary infections in Bangkok ( Table 1 , Supplementary Fig. S2 ). Varying the assumed efficacy of each intervention from 0–100% led to ranges for the estimated contribution of aerosol transmission of ~25–85% in Hong Kong and 25–75% in Bangkok ( Fig. 2 ). Priors and posteriors for the fitted model are shown in Supplementary Figs S3–S4 , and model diagnostics are plotted in Supplementary Figs S5–S8 . Sensitivity analyses with a broad range of alternative model formulations supported these observations ( Supplementary Methods , Supplementary Tables S4–S10 , Supplementary Figs S9–S16 ). 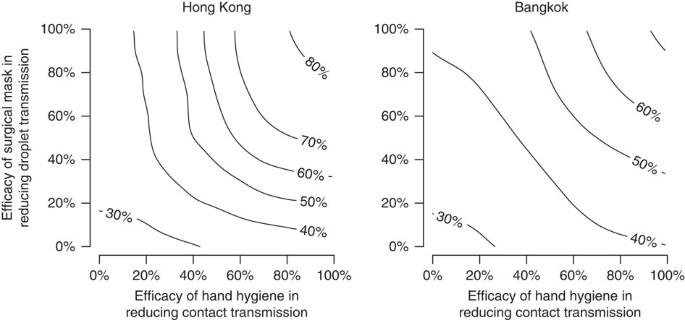Figure 2: The cause-specific probabilities of aerosol transmission. The relative importance of aerosol transmission in households in Hong Kong and Bangkok, quantified in terms of the cause-specific probability of aerosol transmission. The contour lines show the proportion of secondary influenza virus infections attributed to aerosol transmission in the control arm of each study, under varying assumptions about the efficacy of randomization to the hand hygiene and surgical mask interventions in reducing contact (xaxis) and droplet (yaxis) transmission, respectively. The parameter estimates inTable 1correspond to the exemplar plausible assumption that randomization to the hand hygiene and face mask interventions led to 50% reductions in contact and droplet transmission, respectively, from the time of application of those interventions, which corresponds to the centroid of each panel. Figure 2: The cause-specific probabilities of aerosol transmission. The relative importance of aerosol transmission in households in Hong Kong and Bangkok, quantified in terms of the cause-specific probability of aerosol transmission. The contour lines show the proportion of secondary influenza virus infections attributed to aerosol transmission in the control arm of each study, under varying assumptions about the efficacy of randomization to the hand hygiene and surgical mask interventions in reducing contact ( x axis) and droplet ( y axis) transmission, respectively. The parameter estimates in Table 1 correspond to the exemplar plausible assumption that randomization to the hand hygiene and face mask interventions led to 50% reductions in contact and droplet transmission, respectively, from the time of application of those interventions, which corresponds to the centroid of each panel. Full size image Table 1 Parameter estimates for the model of modes of transmission. Full size table Our results suggest that aerosol transmission is an important mode and possibly the predominant mode of influenza A virus transmission in households. Aerosol transmission was estimated to account for approximately half of all transmission events, suggesting that influenza A virus transmission among household members may not be controlled by interventions against contact or droplet transmission [4] , [26] . Our findings were derived from households in tropical and sub-tropical settings but the proposed framework can be used to assess transmission modes in other climates and settings. A comprehensive picture of modes of transmission in different settings would facilitate calibration of public health measures, which only need to reduce overall transmission by approximately one third, assuming a basic reproductive number of ~1.5 (ref. 27 ), to achieve control. Our analysis reveals two important insights into influenza A virus transmission. First, in household outbreaks susceptible individuals are at risk of infection via multiple modes, and substantive reductions in the risk of infection by one mode may not lead to overall reductions in the risk of infection. In the Hong Kong and Bangkok studies, the hand hygiene and face mask interventions did not substantially change the overall risk of infection for household contacts, but instead may have altered the likely mode of infection with consequences for clinical presentation. Second, our model suggests that aerosol transmission appears to be an important mode of transmission in households in Hong Kong and Bangkok, despite previous hypotheses that aerosol transmission may be suppressed in settings with higher humidity [28] , [29] . Whereas other infections that spread predominantly by the aerosol route such as varicella and measles viruses are highly transmissible and can cause explosive outbreaks, influenza viruses are not as highly transmissible, with a reproductive number typically in the range 1.5–2.0 (ref. 27 ). This could be explained if individuals infected with influenza viruses only generate infectious doses at a low rate, so that larger outbreaks would only result from prolonged exposures in optimal conditions [4] , [30] . Assuming that infected persons excrete aerosolized virus at a low rate, and given that infectious virus in aerosols are rapidly diluted through ventilation and natural decay in the environment, it is likely that the greatest risk of aerosol transmission is in close proximity to infected persons [4] . There are some limitations to our analysis. First, our model did not fully account for heterogeneity in transmission associated with various host, viral and environmental factors. For example, there may be variability in infectiousness between index cases, variability in susceptibility to different virus strains and variability in the hazard of modes of transmission depending on proximity and airflow. However, our model captures the essential features of transmission, and random allocation of households to the three intervention arms should have balanced all other factors between groups so that the differences in outcomes between intervention groups are due to the effects of the interventions on modes of transmission. We only included data on influenza A virus transmission in this article because the literature supporting different clinical presentations associated with infections by the aerosol route [22] , [23] only provide data on influenza A. Further work could apply similar approaches to influenza B if the same hypothesis regarding clinical presentation were thought to apply. Second, our model implicitly assumes that only the first infectious exposure is relevant to susceptible contacts, and once infected by that first exposure, further exposures are unimportant. Our model could be expanded to allow for multiple simultaneous exposures, if it were understood how this might affect clinical presentation of consequent infections. Third, it is possible that some secondary influenza virus infections were not confirmed due to poor quality specimens collected during home visits, or if peak viral shedding in the respiratory tract occurred between home visits at 3-day intervals [11] , [12] . Finally, we did not explicitly account for imperfect adherence to the interventions, although the efficacy parameters in our model account for <100% efficacy against the specific modes of transmission as would be expected under imperfect adherence. Further improvements in the model might be obtained by incorporating limited data on adherence that was mainly self-reported by participants. Our results raise a number of questions. First, are there differences in the importance of innate, humoral, cell-mediated and mucosal immunity against specific modes of influenza virus transmission, or in immune responses to infection? Experimental results suggest that humoral antibody might be particularly relevant for protection against aerosol transmission [22] . Second, are there differences in the incubation period associated with infection by different modes of transmission? It is thought that the minimum infectious dose is lower for infections by the aerosol route [22] , [23] , but the implications on incubation period are unclear. Third, are there consequences from the mode of infection on modes of subsequent transmission from an infected and symptomatic (or asymptomatic) individual? If so, there would be important implications for the interpretation of volunteer challenge and transmission studies? [31] Finally, how would repeated exposures to infectious doses of influenza viruses, particularly within a short time frame after the first exposure, affect subsequent risk of clinical disease and clinical presentation? As some genetic factors have been identified as risk factors for severe influenza disease [32] , [33] , what is the role of such factors in influencing milder clinical diseases versus no illness by different modes of influenza virus transmission? Further work could examine differences in modes of influenza virus transmission by host, viral and environmental factors, in other geographical locations, and in other closed environments including schools and health care settings. In particular, there is some evidence that absolute humidity influences aerosol transmission [28] , [29] , [34] , and our results lead to the corollary that the clinical presentation of influenza virus infections could vary over time according to variation in humidity. On the technical side, further work could explore the use of alternative modelling approaches including dependent competing risk models. In conclusion, our findings suggest that household contacts of persons with symptomatic influenza virus infection are at risk of infection by multiple modes, and that aerosol transmission is important. This is suggestive of the need for further studies into personal preventive measures for the control of influenza; although our observations suggest that hand hygiene and surgical face masks may not provide high levels of protection against influenza virus transmission in these settings. Having identified that aerosol transmission is important in households, appropriate control measures in this setting could include improved ventilation to dilute and remove aerosols more quickly, the use of humidifiers or ultraviolet light to reduce the viability of aerosols and isolation of sick individuals in separate rooms [26] , [28] . The importance of aerosol transmission implies that the definition of ‘contact’ in epidemiological studies of influenza virus transmission may need to be reconsidered, perhaps by accounting for proximity and duration of contact. Although our findings offer new insights in understanding and preventing influenza transmission in a confined space, the relative contribution of each mode of transmission has yet to be clarified in other geographical locations and different transmission settings. Our model also enables more detailed analyses of the effects of host factors (for example, age, innate, humoral and mucosal immunity), differences between virus strains, and environmental factors (temperature, humidity, air currents) in varying the importance of each mode of transmission. Sources of data In Hong Kong and Bangkok during 2008–2011, large randomized controlled trials were conducted to investigate the efficacy of surgical face masks and enhanced hand hygiene in reducing transmission of influenza in households [11] , [12] . The two studies shared very similar protocols as outlined below, and minor differences between the two studies are clarified in Supplementary Table S11 . In each study, index cases were enrolled as local residents presenting for medical care with illness consistent with an acute upper respiratory tract infection, and living in a household with at least two other individuals of whom none had reported upper respiratory tract infections in the preceding 14 days. Nasal and throat swabs (NTS) were collected and pooled for testing with the QuickVue Influenza A+B rapid diagnostic test (Quidel Corp., San Diego, CA) using the manufacturer’s sterile foam swabs. Those subjects with a positive result on the rapid test were randomized and further followed-up. Data on clinical signs and symptoms were collected for all subjects, and an additional pooled NTS specimen was collected for subsequent reference testing. Households were randomized in equal proportions to one of three groups: control, control plus hand hygiene or control plus hand hygiene plus surgical face masks. Supplementary Table S12 provides specific details of the three interventions applied in each study. Following randomization a home visit was scheduled to implement the intervention, collect baseline demographic data and NTS specimens from all household members aged ≥2 years, and to describe the information to be recorded in daily symptom diaries. Further home visits were scheduled around 3 and 6 days after the baseline home visit to check symptom diaries, monitor adherence to interventions and collect NTS specimens from all household members regardless of illness. All NTS specimens were tested by RT–PCR for influenza A and B viruses using standard methods as described elsewhere [7] , [8] . Only the households of index cases with confirmed influenza A virus infection are included in the present analyses. The primary outcome measure was the secondary infection risk at the individual level, that is, the proportion of household contacts that had influenza virus infection confirmed by RT–PCR during follow-up. Written informed consent was provided by all subjects 18 years of age and older, and proxy written consent from parents or legal guardians was obtained for children. The studies were approved by Institutional Review Boards in Hong Kong and Bangkok, respectively. Statistical analysis We constructed a mathematical model that accounted for the alternative modes of transmission ( Supplementary Methods , Supplementary Tables S13–S15 , Supplementary Fig. S17 ) and used it to analyse the observed time intervals between primary and secondary cases, the frequency of secondary transmission in households and the risk of presentation with fever plus cough among confirmed secondary cases. As the observation of household transmission was truncated at around 7 days as illness onset in each index case, we assumed that all of observed secondary cases resulted from actual secondary transmission. We estimated the cumulative hazards of infection with or without fever in each study arm using the Nelson–Aalen non-parametric estimator. Using the competing risk model described in the Supplementary Information , we allowed household contacts to experience competing hazards of infection by three alternative modes, and time to infection in each mode followed a Weibull distribution with an identical shared shape parameter and mode-specific scale parameters. Infection via one mode was sufficient to confer immunity against any further infection. In households with one or more secondary case, we assumed independent hazards of infection from each infected person in a household for the remaining contacts. Some household contacts were assumed to be immune to infection by any mode, and we jointly estimated the proportion of initially immune children and adults with other parameters. We assumed that randomization to the hand hygiene intervention reduced the risk of contact transmission, and the addition of surgical face masks also reduced the risk of droplet transmission independently. Moreover, we assumed a different risk of fever plus cough following infection with each mode of transmission. Quantifying each hazard of secondary transmission, we computed the cause-specific probability of aerosol transmission to express the relative contribution of aerosol transmission among all three modes. Data from the Hong Kong study and statistical syntax in the R language to permit reproduction of these analyses are available at the corresponding author’s website ( http://www.hku.hk/bcowling/influenza/HK_NPI_study.htm ). How to cite this article: Cowling, B. J. et al . Aerosol transmission is an important mode of influenza A virus spread. Nat. Commun. 4:1935 doi: 10.1038/ncomms2922 (2013).